A poly(A)-specific ribonuclease directly regulates the poly(A) status of mitochondrial mRNA inArabidopsis Coordination of gene expression in the organelles and the nucleus is important for eukaryotic cell function. Transcriptional and post-transcriptional gene regulation in mitochondria remains incompletely understood in most eukaryotes, including plants. Here we show that poly(A)-specific ribonuclease, which influences the poly(A) status of cytoplasmic mRNA in many eukaryotes, directly regulates the poly(A) tract of mitochondrial mRNA in conjunction with a bacterial-type poly(A) polymerase, AGS1, in Arabidopsis . An Arabidopsis poly(A)-specific ribonuclease-deficient mutant, ahg2-1 , accumulates polyadenylated mitochondrial mRNA and shows defects in mitochondrial protein complex levels. Mutations of AGS1 suppress the ahg2-1 phenotype. Mitochondrial localizations of AHG2 and AGS1 are required for their functions in the regulation of the poly(A) tract of mitochondrial mRNA. Our findings suggest that AHG2 and AGS1 constitute a regulatory system that controls mitochondrial mRNA poly(A) status in Arabidopsis . Mitochondria and plastids (in plants) are genome-harbouring symbiotic organelles. Coordinated expression of organelle genome-encoded and nuclear genome-encoded genes is fundamental to a range of cellular processes in eukaryotes [1] , [2] . Although mitochondrial functions are conserved among eukaryotes, genome structure and the regulatory mechanisms for gene expression in mitochondria are, surprisingly, quite divergent [3] . Plants are unique in that they possess extremely large mitochondrial genomes [4] and exhibit complex mechanisms for editing mitochondrial mRNA [5] , [6] involving a large family of pentatricopeptide repeat proteins [7] , [8] . Presumably due to their sessile lifestyle and/or the presence of plastids, regulation of mitochondrial gene expression appears to be quite important for plants. However, the molecular basis of gene regulation in plant mitochondria is not fully understood [9] , [10] . The quality and quantity of various types of RNA molecules are surveyed and regulated by a so-called RNA quality control system [11] , [12] , [13] . The polyadenine (poly(A)) tract added to the 3′ end of a RNA molecule has a pivotal role in RNA quality control. The poly(A) tract of cytoplasmic mRNA is mainly regulated by two types of enzymes, poly(A) polymerases (PAP) and deadenylases, including the CCR4–NOT complex, the PAN2–PAN3 complex and poly(A)-specific ribonuclease (PARN) [14] , [15] . Organellar mRNA is also subject to the control of stability. However, the physiological relevance of polyadenylation and the regulatory mechanisms acting on the poly(A) tract in organelles are different among organisms, and their regulatory systems are not fully understand in most organisms [9] , [16] , [17] , [18] . Arabidopsis possesses one gene encoding a functional PARN, named AHG2 (also known as AtPARN) [19] , [20] , [21] . Plants harbouring a weak mutant allele of this gene display a dwarf phenotype and respond abnormally to the stress-related phytohormones abscisic acid (ABA) and salicylic acid (SA) [21] , [22] . Null mutants are not viable [19] , [20] , [21] , suggesting that AHG2 has an important and unique function in Arabidopsis . Here we show that AHG2, in cooperation with a bacterial-type PAP named AGS1, regulates mitochondrial mRNA by affecting the poly(A) tract, which acts as a degradation tag. We found that the Arabidopsis ahg2-1 (ref. 21 ) mutant deficient in PARN accumulates polyadenylated mitochondrial mRNA, whereas wild type and ahg2-1 suppressor mutants ( ags1 ; defective in AGS1) do not. We demonstrate that the levels of mitochondrial protein complexes are disturbed in ahg2-1 , and that mitochondrial localization of AHG2 and AGS1 are required for their functions in the regulation of the poly(A) tract of mitochondrial mRNA. We propose a model in which AHG2 and AGS1 constitute a regulatory system that controls mitochondrial mRNA poly(A) status in Arabidopsis and postulate that plants have co-opted the cytosolic mRNA regulator PARN for use as a mitochondrial regulator. ags1 suppresses the phenotype of PARN-deficient mutants To address the physiological function of AHG2, genetic screening for ahg2-1 suppressor mutants was conducted. The ahg2-1 mutant has short roots, a phenotype that could not be rescued by abscisic acid ( abi3 , abi5 and aba2 )- or salicylic acid ( eds1 and pad4 )-deficient mutants. Using the root elongation rate as a phenotypic marker, eight putative suppressor mutants for ahg2-1 (termed ags for a h g 2-1 s uppressor ) were isolated ( Fig. 1a ). Most of the ags mutants had normal-sized shoots and leaves, and a normal ABA response at germination in the ahg2-1 mutant background ( Fig. 1b,c , Supplementary Fig. S1a ). The endogenous SA levels and bacterial growth inhibition on the true leaves, which are higher in ahg2-1 than in the wild type, were strongly reduced in the ags mutants ( Supplementary Fig. S1b,c ). Taken together, our findings show that the ags mutations restore all of the known ahg2-1 phenotypes, implying that the molecular functions affected by these suppressor mutations are closely related to AHG2 function. 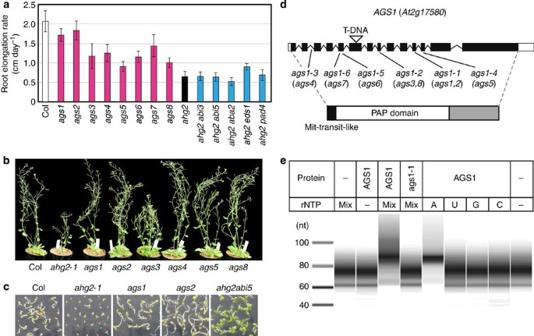Figure 1: Theahg2-1 suppressorgene encodes a poly(A) polymerase. (a) Elongation rate of the primary root. The root elongation rates ofahg2-1 suppressorcandidates (sup), wild type,ahg2-1and double mutants ofahg2-1and abscisic acid (abi3, abi5andaba2)- or salicylic acid (eds1andpad4)-deficient mutants are shown. Error bars indicate s.d. (n>10). (b) Phenotype of aerial parts of 5-week-old wild-type,ahg2-1andahg2-1 suppressormutant plants. (c) Response to ABA during germination. Stratified seeds of indicated lines were sown on agar plates containing 0.3 μM ABA and incubated for 5 days. (d) The predicted gene structure ofAGS1.The mutation sites of established suppressor mutants are indicated. The predicted overall protein structure is also shown. (e) Polymerase activity of recombinant AGS1 proteinsin vitro. Recombinant AGS1 or ags1-1 protein was incubated with a template RNA and ribonucleotides (rNTP; mixture of four ribonucleotides, or each ribonucleaotide alone as indicated) and analysed by capillary electrophoresis. ‘–’ indicates no addition. Capillary RNA electrophoresis patterns are shown with a size maker. Figure 1: The ahg2-1 suppressor gene encodes a poly(A) polymerase. ( a ) Elongation rate of the primary root. The root elongation rates of ahg2-1 suppressor candidates ( sup ), wild type, ahg2-1 and double mutants of ahg2-1 and abscisic acid ( abi3, abi5 and aba2 )- or salicylic acid ( eds1 and pad4 )-deficient mutants are shown. Error bars indicate s.d. ( n >10). ( b ) Phenotype of aerial parts of 5-week-old wild-type, ahg2-1 and ahg2-1 suppressor mutant plants. ( c ) Response to ABA during germination. Stratified seeds of indicated lines were sown on agar plates containing 0.3 μM ABA and incubated for 5 days. ( d ) The predicted gene structure of AGS1. The mutation sites of established suppressor mutants are indicated. The predicted overall protein structure is also shown. ( e ) Polymerase activity of recombinant AGS1 proteins in vitro . Recombinant AGS1 or ags1-1 protein was incubated with a template RNA and ribonucleotides (rNTP; mixture of four ribonucleotides, or each ribonucleaotide alone as indicated) and analysed by capillary electrophoresis. ‘–’ indicates no addition. Capillary RNA electrophoresis patterns are shown with a size maker. Full size image Map-based cloning revealed ags1 to be At2g17580 . Interestingly, all of the other sup mutants also harboured a mutation in this gene ( Fig. 1d ). Hereafter, we termed this gene AGS1 and numbered the ags mutants as shown in Fig. 1d . AGS1 encodes a protein with a bacterial-type poly(A) polymerase domain. A mitochondrial transit peptide-like sequence was detected at its N terminus. All mutations appeared likely to reduce PAP activity, either by altering amino-acid residues that are conserved among PAPs or by causing production of a truncated polypeptide ( Supplementary Fig. S2 ), suggesting that ags1 mutations lead to loss-of-function effects. Supporting this idea, recombinant AGS1 protein had polymerase activity with a strong preference for adenine, whereas recombinant ags1-1 mutant protein displayed no activity ( Fig. 1e ), and a T-DNA insertion knockout mutation of AGS1 (SALK_083725) also could rescue ahg2-1. Homozygous ags1-1 could suppress the lethality of the AHG2- knockout mutation, although growth was still partially compromised ( Supplementary Fig. S3a,b ), suggesting that at least this suppressor mutant is not allele-specific. Analysis of genomic data indicated that Arabidopsis has several bacterial-type PAPs, and one of these has been shown to possess PAP activity [23] . The isolation of only ags1 mutants in our screen for ahg2-1 suppressors implies that AGS1 has a specific function not shared with the other PAPs in Arabidopsis . As ags1 heterozygotes could suppress the ahg2-1 phenotype, ags1 mutations appeared to be dominant. However, transgenic expression of ags1-1 did not suppress the ahg2-1 phenotype of ahg2-1 AGS1 plants, whereas expression of wild-type AGS1 counteracted the suppressor effects of ags1 . Monogenic ags1 lines showed no detectable phenotypes. Thus, an imbalance between AHG2 and AGS1 activities, viz., relatively less AHG2 activity compared with AGS1, appears to underlie the ahg2-1 phenotype. Polyadenylated mitochondrial mRNA is accumulated in ahg2-1 The data described above suggested that changes in the poly(A) status of certain RNA(s) are responsible for the ahg2-1 phenotype. As PARN in other organisms is involved in the degradation of cytoplasmic mRNA by removing the poly(A) tract, we first postulated that the target RNAs of AHG2 would be nuclear-encoded cytoplasmic mRNAs, and that they should be accumulated markedly and have a longer poly(A) tail in ahg2-1 . As we previously reported, the transcripts of dozens of nuclear-encoded genes accumulated specifically in ahg2-1 (ref. 21 ). However, we failed to detect longer poly(A) tracts of those transcripts in ahg2-1 . A genomic tiling array analysis did not reveal any novel transcripts to be highly accumulated in ahg2-1 ( Supplementary Table S1 ). Intriguingly, the ahg2-1 array experiments consistently displayed high mitochondrial mRNA levels [22] . We then conducted poly(A)-tail (PAT) assays for mitochondrial cox1 , cox2 , orf107f , nad7 and atp9 transcripts and found that DNA fragments could be amplified from the ahg2-1 cDNA sample, but not from the wild-type and ags1 mutant cDNA samples ( Fig. 2a,b ) [24] . Sequencing analysis revealed that these DNA fragments indeed had poly(A) tracts at the positions proximal to the reported 3′ ends of these mitochondrial mRNAs [25] . Moreover, the nad7 PAT DNA fragment exhibited RNA editing as previously reported [26] . These data strongly suggested that these amplified poly(A)-DNA fragments originated from mitochondrial mRNA. Circularization RT–PCR (cRT–PCR) experiments revealed that about half of the investigated transcripts in ahg2-1 possessed poly(A) sequences, ranging from a few to 20 nucleotides, immediately downstream of the 3′-end ( Fig. 2c,d , Supplementary Table S2 ). We previously reported that ahg2-1 shares several characteristics, such as the gene expression profile, ABA hypersensitivity and dwarf phenotype, with an AtPHB3 T-DNA insertion mutant, atphb3 , which was reported to exhibit mitochondrial dysfunction [22] . However, poly(A) tracts were not detected in mitochondrial mRNA in atphb3 ( Fig. 2b ), suggesting strongly that mitochondrial dysfunction is not the cause of the accumulation of polyadenylated mitochondrial mRNA in ahg2-1 . 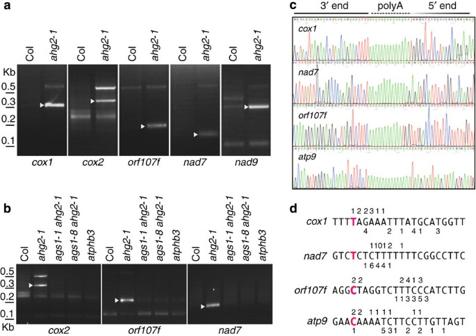Figure 2: Theahg2-1mutation causes accumulation of poly(A)+mitochondrial mRNA. (a,b) PAT assays for transcripts of the indicated mitochondrial genome-encoded genes in wild type (Col) andahg2-1(a) and in suppressor mutants oratphb3(b). Arrowheads indicate PAT products. (c) Representative poly(A) structures of mitochondrial mRNA inahg2-1detected by cRT–PCR. (d) Summary of the positions of polyadenylation. Red-coloured residues represent the end of the mRNA as deduced from wild-type cRT–PCR products and from a previous report25. The number above or under each residue indicates the number of clones ending or polyadenylated at this position, respectively. Figure 2: The ahg2-1 mutation causes accumulation of poly(A) + mitochondrial mRNA. ( a , b ) PAT assays for transcripts of the indicated mitochondrial genome-encoded genes in wild type (Col) and ahg2-1 ( a ) and in suppressor mutants or atphb3 ( b ). Arrowheads indicate PAT products. ( c ) Representative poly(A) structures of mitochondrial mRNA in ahg2-1 detected by cRT–PCR. ( d ) Summary of the positions of polyadenylation. Red-coloured residues represent the end of the mRNA as deduced from wild-type cRT–PCR products and from a previous report [25] . The number above or under each residue indicates the number of clones ending or polyadenylated at this position, respectively. Full size image Levels of mRNA and protein complexes in ahg2-1 mitochondria To obtain more insight into the mitochondrial phenotype in ahg2-1 , mitochondria were visualized using Mt-GFP [27] in ahg2-1 and wild-type plants or protoplasts. Microscopic observations did not reveal any obvious difference in the number or shape of mitochondria between the samples ( Fig. 3a ). Next, the relative amount of mitochondrial genome DNA (mt-DNA) to nuclear genome DNA (nc-DNA) was deduced using qPCR analyses of the mitochondrial-encoded genes cox2 and nad4 and the nuclear-encoded gene AGS1 . The ahg2-1 plants were found to have an ~1.5-fold higher mt-DNA:nc-DNA ratio than wild-type plants. Recent studies have shown that mt-DNA level per mitochondrion varies significantly among tissues and cell types in plants [28] , [29] . To test whether the ahg2-1 mutation indirectly affects mt-DNA level per mitochondrion, we examined DNA and mRNA levels in mitochondria purified from ahg2-1 or wild-type cultured cells. The mt-DNA level per mitochondrion was estimated by qPCR analyses for cox2 and nad4 normalized to total mitochondrial protein levels. As shown in Fig. 3b , the mt-DNA level per mitochondrion did not significantly differ between the ahg2-1 and wild-type mitochondria. In light of the increased mt-DNA:nc-DNA ratio in ahg2-1 , this result suggests that the mitochondrial volume (per nc-DNA) increased ~1.5-fold in ahg2-1 , based on the assumption that the protein level reflects mitochondrion volume. The mitochondrial mRNA levels were estimated by RT–qPCR analyses for cox2 and nad4 normalized to mt-DNA levels. Interestingly, they were ~1.5-fold higher in ahg2-1 mitochondria than in wild-type mitochondria. Taken together, both the mitochondrial volume and mitochondrial mRNA levels (per nc-DNA) were increased in ahg2-1 . Consistent with these data, RNA gel blot analyses for mitochondrial-encoded genes showed that mRNA levels increased in ahg2-1 ; the increment varied among genes from 1.3- to 4-fold. The RNA gel blot analyses also revealed that the length of each transcript was not different between ahg2-1 and wild type ( Fig. 3c ). The RNA editing status of nad7 was examined by sequencing dozens of cDNA clones, but no significant abnormalities were detected. These data suggest that ahg2-1 affects poly(A) status and levels, but not splicing or editing, of mRNA in mitochondria. 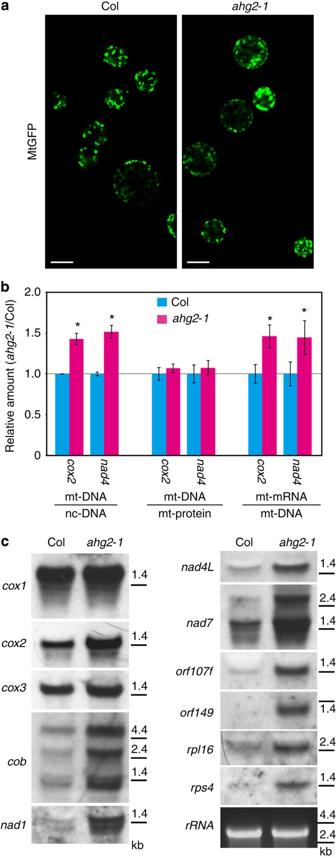Figure 3: Theahg2-1mutation affects mitochondrial RNA levels. (a) Microscopic observation of Mt-GFP in wild type andahg2-1.Arabidopsisprotoplasts were obtained from wild-type andahg2-1plants harbouring the MtGFP gene. Scale bars indicate 20 μm. (b) Relative amounts of mt-DNA to genomic DNA, mt-DNA to mitochondrial protein and mitochondrial mRNA to mt-DNA. Total DNA prepared from 2-week-old plants was used for qPCR analysis of mitochondrial-encodedcox2andnad4, and of nuclear-encodedAGS1, and the relative amount of mt-DNA to nc-DNA was deduced. Using mt-DNA or mRNA isolated from wild-type orahg2-1mitochondria preparations, relative mt-DNA or mRNA levels for each gene were deduced by qPCR analysis (for DNA) normalized to the total mitochondrial protein levels or RT–qPCR analysis (for mRNA) normalized to the deduced mt-DNA levels. Averages with standard deviations of the data obtained using three total DNA preparations and three independent mitochondria preparations are shown. *P-values <0.05 by Student’st-tests betweenahg2-1and wild-type (Col) lines. Error bars indicate s.d. (n=3). (c) RNA gel blotting of mitochondrial mRNA. Total RNA was prepared from 3-week-old plants. rRNA was used as loading control. Figure 3: The ahg2-1 mutation affects mitochondrial RNA levels. ( a ) Microscopic observation of Mt-GFP in wild type and ahg2-1 . Arabidopsis protoplasts were obtained from wild-type and ahg2-1 plants harbouring the MtGFP gene. Scale bars indicate 20 μm. ( b ) Relative amounts of mt-DNA to genomic DNA, mt-DNA to mitochondrial protein and mitochondrial mRNA to mt-DNA. Total DNA prepared from 2-week-old plants was used for qPCR analysis of mitochondrial-encoded cox2 and nad4 , and of nuclear-encoded AGS1 , and the relative amount of mt-DNA to nc-DNA was deduced. Using mt-DNA or mRNA isolated from wild-type or ahg2-1 mitochondria preparations, relative mt-DNA or mRNA levels for each gene were deduced by qPCR analysis (for DNA) normalized to the total mitochondrial protein levels or RT–qPCR analysis (for mRNA) normalized to the deduced mt-DNA levels. Averages with standard deviations of the data obtained using three total DNA preparations and three independent mitochondria preparations are shown. * P -values <0.05 by Student’s t -tests between ahg2-1 and wild-type (Col) lines. Error bars indicate s.d. ( n =3). ( c ) RNA gel blotting of mitochondrial mRNA. Total RNA was prepared from 3-week-old plants. rRNA was used as loading control. Full size image Mitochondrial protein levels were assessed using mitochondria purified from cultured wild-type or ahg2-1 cells. Immunoblotting revealed that the cox2 and nad9 levels of ahg2-1 mitochondria were higher than those of the wild-type mitochondria whereas the levels of nuclear genome-encoded proteins did not differ significantly between these plants ( Fig. 4a , ahg2-1 :wild-type signal intensity ratios were cytc, 1.05; SDH1, 1.28; αMPP, 0.90; βSUB, 1.21; cox2, 7.58; nad9, 2.42). Blue-native (BN)–PAGE of mitochondrial extracts showed different banding patterns in wild type and ahg2-1 ( Fig. 4b ). Immunoblotting with anti-αMPP antibody ( Fig. 4c ) revealed that the major missing band in ahg2-1 corresponded to complex III, which is a major ROS producer in both animal and plant cells [30] , [31] . On the other hand, anti-cox2 blotting indicated higher complex IV levels ( Fig. 4c ). These results suggest that increased mitochondrial mRNA levels result in the accumulation of their translational products in ahg2-1 , which, in turn, might compromise the stability of the mitochondrial protein complexes, presumably due to the disturbed stoichiometry among nuclear-encoded and mitochondrial-encoded complex components, as observed in animal or yeast mitochondria [32] . 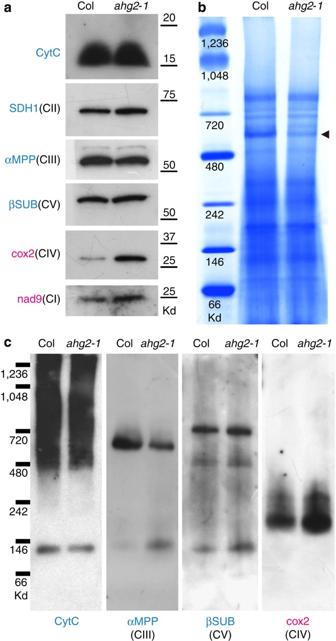Figure 4: Theahg2-1mutation affects mitochondrial protein and protein complex levels. (a,b) Immunoblotting of mitochondrial proteins separated by SDS–PAGE (a) or by BN–PAGE (c). Protein names in blue or red indicate nuclear- or mitochondrial-encoded protein, respectively. (b) BN–PAGE of mitochondrial proteins. The arrowhead indicates the band corresponding to complex III. Figure 4: The ahg2-1 mutation affects mitochondrial protein and protein complex levels. ( a , b ) Immunoblotting of mitochondrial proteins separated by SDS–PAGE ( a ) or by BN–PAGE ( c ). Protein names in blue or red indicate nuclear- or mitochondrial-encoded protein, respectively. ( b ) BN–PAGE of mitochondrial proteins. The arrowhead indicates the band corresponding to complex III. Full size image AHG2 and AGS1 localize to and function in mitochondria To examine the subcellular localization of AHG2 and AGS1, we constructed translational fusions between their genomic sequences and the reporter gene GFP. The genomic DNA fragments of these genes, including part of the upstream or downstream proximal gene, were cloned and the GFP gene was inserted in-frame near the stop codon. Using these recombinant genes, several transgenic Arabidopsis lines were established. For both genes, strong GFP fluorescence was detected in root and shoot primordia and weak fluorescence was observed throughout the plant. GFP signal in the AHG2–GFP transgenic plants completely colocalized with MitoTracker Red signal ( Fig. 5a ). In AGS1–GFP transgenic plants, GFP signals partly overlapped with MitoTracker signals, but also localized to the nuclei in cells with presumably higher proliferation activity ( Fig. 5b , Supplementary Fig. S4 ). In addition, immunoblotting with an anti-GFP antibody showed that GFP fusion proteins were exclusively in the mitochondrial fraction ( Supplementary Fig. S5 ). Recently, AHG2 was reported to localize at cytoplasmic foci. The discrepancy in the subcellular localization of AHG2 can be due to the difference in the experimental systems; our study used stable transgenic plants harbouring the AHG2–GFP fusion gene generated from the full-length genomic sequence including the putative promoter region, while Moreno et al . [33] expressed a fusion gene with the truncated AHG2 genomic sequence under 35S promoter in a transient expression system using tobacco plants. Our data here indicated that AHG2 and AGS1 proteins preferentially localize to mitochondria, and implied that the subcellular localization of AGS1 protein could be regulated by developmental or cellular physiological status. 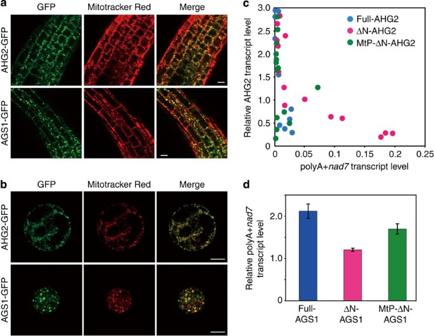Figure 5: AHG2 and AGS1 localize to mitochondria. (a) Localization of AHG2-GFP and AGS1-GFP inArabidopsisroots. Roots of transgenic plants harbouring genomicAHG2orAGS1sequences fused in-frame to theGFPgene were stained with MitoTracker Red. Scale bars indicate 10 μm. (b) Subcellular localization of AHG2–GFP and AGS1–FP inArabidopsisroot protoplasts obtained from the transgenic plants stained with Mitotracker Red. Scale bars indicate 10 μm. (c,d) Effect of the removal of the putative transit peptide from the AHG2 and AGS1 N-terminal regions. (c) Relative levels of polyadenylatednad7transcript inahg2-1transgenic plants harbouring the35 Spromoter-driven wild-type (Full-AHG2), ΔN– or MtP–ΔN–AHG2genes. The levels of polyadenylatednad7transcript were deduced by RT–qPCR fornad7PAT DNA andACT2.xaxis: relative levels of recombinantAHG2transcript in transgenic plant normalized toACT2.yaxis: relative levels of polyadenylatednad7transcript in transgenic plants normalized to theACT2levels. Each dot point represents one transgenic plant. (d) Relative levels of polyadenylatednad7transcript in wild-type mesophyll protoplasts transfected with the35 Spromoter-driven wild-type, ΔN- or MtP–ΔN–AGS1genes.35S–GFPwas used to monitor the transfection efficiencies (~80%) and also as a negative control. PAT assays fornad7transcripts were conducted using RNA samples derived from transfected protoplasts. PAT DNA levels were measured from fluorescence of the DNA bands in agarose gels (Supplementary Fig. S6) and were normalized to theACT2levels detected by RT–qPCR. Then the amounts relative to the background levels inGFP-transfected protoplasts were calculated. The average of the relative polyadenylatednad7transcript levels with standard deviation obtained from three independent transfection assays is shown. Figure 5: AHG2 and AGS1 localize to mitochondria. ( a ) Localization of AHG2-GFP and AGS1-GFP in Arabidopsis roots. Roots of transgenic plants harbouring genomic AHG2 or AGS1 sequences fused in-frame to the GFP gene were stained with MitoTracker Red. Scale bars indicate 10 μm. ( b ) Subcellular localization of AHG2–GFP and AGS1–FP in Arabidopsis root protoplasts obtained from the transgenic plants stained with Mitotracker Red. Scale bars indicate 10 μm. ( c , d ) Effect of the removal of the putative transit peptide from the AHG2 and AGS1 N-terminal regions. ( c ) Relative levels of polyadenylated nad7 transcript in ahg2-1 transgenic plants harbouring the 35 S promoter-driven wild-type (Full-AHG2), ΔN– or MtP–ΔN– AHG2 genes. The levels of polyadenylated nad7 transcript were deduced by RT–qPCR for nad7 PAT DNA and ACT2 . x axis: relative levels of recombinant AHG2 transcript in transgenic plant normalized to ACT2 . y axis: relative levels of polyadenylated nad7 transcript in transgenic plants normalized to the ACT2 levels. Each dot point represents one transgenic plant. ( d ) Relative levels of polyadenylated nad7 transcript in wild-type mesophyll protoplasts transfected with the 35 S promoter-driven wild-type, ΔN- or MtP–ΔN– AGS1 genes. 35S – GFP was used to monitor the transfection efficiencies (~80%) and also as a negative control. PAT assays for nad7 transcripts were conducted using RNA samples derived from transfected protoplasts. PAT DNA levels were measured from fluorescence of the DNA bands in agarose gels ( Supplementary Fig. S6 ) and were normalized to the ACT2 levels detected by RT–qPCR. Then the amounts relative to the background levels in GFP- transfected protoplasts were calculated. The average of the relative polyadenylated nad7 transcript levels with standard deviation obtained from three independent transfection assays is shown. Full size image To confirm the mitochondrial function of AHG2 and AGS1, we tested whether their putative N-terminal transit sequences were required for their functions. Recombinant proteins in which the putative N-terminal transit peptides of these proteins were removed (ΔN−) or replaced with the known functional mitochondrial transit sequence of At5g14580 (MtP–ΔN−) [23] were expressed under a cauliflower mosaic virus 35S promoter in ahg2-1 plants, or in wild-type mesophyll protoplast cells ( Supplementary Fig. S6 ). As shown in Fig. 5c , wild-type AHG2 and MtP–ΔN–AHG2 efficiently reduced the polyadenylated nad7 transcript levels, even in transgenic lines with lower transgene expression levels. By contrast, ΔN–AHG2 was less effective in reducing the polyadenylated nad7 transcript levels in plants with lower transgene expression levels. Presumably, the AHG2 N-terminal sequence is not the sole determinant of its mitochondrial localization, because ΔN–AHG2 could be localized to mitochondria in plants ( Supplementary Fig. S6 ). Although removing the N-terminal portion of the protein did not prevent mitochondrial localization completely, it resulted in decreased polyadenylated nad7 transcript levels in line with high ΔN–AHG2 expression. The necessity of mitochondrial localization for AGS1 function was also demonstrated. As shown in Fig. 5d , polyadenylated nad7 transcript accumulated markedly in protoplasts transfected with wild-type AGS1 and MtP–ΔN–AGS1, but did not accumulate in those transfected with ΔN–AGS1. These data indicated that AHG2 and AGS1 localize to and function within mitochondria to regulate the poly(A) status of mitochondrial mRNA. We next expressed AGS1 proteins in budding yeast cells, where polyadenylation of mitochondrial mRNA has not previously been observed, and examined their activity. AHG2–GFP yielded a fluorescent signal both in mitochondria and the cytoplasm, whereas AGS1–GFP exhibited a strong signal in mitochondria in yeast cells ( Supplementary Fig. S7 ), suggesting that these proteins localize to mitochondria in yeast cells as well as in plant cells. We transformed yeast cells with plasmids bearing recombinant genes, and performed a PAT assay for yeast COX3 transcripts. Expression of AGS1, but not ags1-1 or ΔN–AGS1, resulted in the accumulation of polyadenylated COX3 transcripts ( Supplementary Fig. S7 ), consistent with the data shown above ( Figs 1e and 4d ). These results suggest that AGS1 alone can regulate the poly(A) status of mRNA in a heterologous mitochondrial system. Co-expressing AHG2 with AGS1 in budding yeast did not have any effects on the addition of poly(A) by AGS1. It is possible that AHG2 function requires additional factors. In this study, we demonstrated that a defect in a poly(A) polymerase of Arabidopsis , named AGS1, suppresses all of the known phenotypes of the PARN-deficient mutant ahg2-1 . This indicates that an imbalance between the addition and removal of polyadenylation in certain RNAs causes the ahg2-1 phenotype. We searched for the target RNAs of AHG2 by analysing transcript levels and their poly(A) status in ahg2-1 , and unexpectedly found that ahg2-1 uniquely accumulates polyadenylated mitochondrial mRNA. This molecular phenotype was completely suppressed by ags1-1 or ags1-8, suggesting that AHG2 and AGS1 are involved in the regulation of poly(A) tracts of mitochondrial mRNA either directly or indirectly. The mitochondrial localizations of these proteins were assessed using transgenic plants carrying the AHG2–GFP or AGS1–GFP gene whose expression was driven by the native promoter. In addition, the putative N-terminal transit peptides of both proteins were required for their functions in the regulation of the poly(A) tract of mitochondrial mRNA. Together, these results strongly suggest that AGS1 and AHG2 regulate the poly(A) status of mitochondrial mRNA in Arabidopsis . As reported previously, mutations disrupting AHG2 are embryonic lethal [19] , [20] , [21] , and ahg2-1 causes hypersensitivity to the phytohormones ABA and SA [21] , demonstrating that the defect in AHG2 compromises fundamental cellular functions of plants. Based on all of these data, we propose that plants have a unique system for regulating mitochondrial gene expression, in which AGS1 (PAP) and AHG2 (PARN) control mRNA stability through regulating poly(A) status in mitochondria ( Fig. 6 ). Perturbation of the AGS1–AHG2 system leads to dysfunctional mitochondria, which, in turn, has harmful effects on various cellular functions, causing embryonic death or abnormal responses to stress-related plant hormones as observed in the ahg2 mutants. Thus, this system has a pivotal role in the coordination between mitochondrial and cellular functions. In plant mitochondria, polyadenylated mitochondrial mRNA is believed to be degraded immediately. Based on current knowledge, PARN has deadenylase activity but not broad substrate-specific exonuclease activity. Previous reports showed that recombinant Arabidopsis PARN/AHG2 proteins degrade only the poly(A) tract during in vitro assays [21] , [19] . Accumulation of polyadenylated mitochondrial mRNA in ahg2-1 implies that AHG2 is also involved in the degradation of mRNA in mitochondria. The removal of the poly(A) tract by AHG2 might trigger degradation of the mRNA. Alternatively, AHG2 might recruit the RNA degradation machinery to the mRNA. A polynucleotide phosphorylase (PNPase) was previously shown to have a role in the control of mRNA stability in mitochondria [34] . The PNPase-defective lines exhibited accumulation of by-product RNAs, which is not observed in the ahg2-1 mutant, suggesting that PARN and PNPase function in different ways. 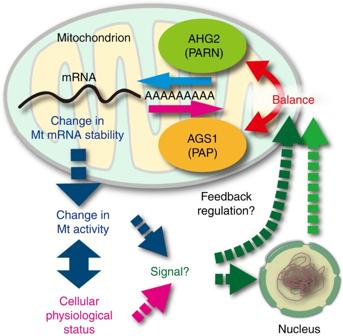Figure 6: Proposed model of AHG2 and AGS1 functions in the plant stress response. In this model, AHG2 and AGS1 constitute a regulatory system for the maintenance of mitochondrial mRNA levels in response to cellular physiological status. Our data indicated that the balance between AHG2 and AGS1 directly affects the poly(A) status of mRNA in plant mitochondria, where poly(A) signals function as a degradation tag. Disruption of this balance impairs mitochondrial function and cellular activities, including stress-related hormonal responses. Figure 6: Proposed model of AHG2 and AGS1 functions in the plant stress response. In this model, AHG2 and AGS1 constitute a regulatory system for the maintenance of mitochondrial mRNA levels in response to cellular physiological status. Our data indicated that the balance between AHG2 and AGS1 directly affects the poly(A) status of mRNA in plant mitochondria, where poly(A) signals function as a degradation tag. Disruption of this balance impairs mitochondrial function and cellular activities, including stress-related hormonal responses. Full size image In plants, ABA and SA have pivotal roles in abiotic and biotic stress responses, respectively, and their signalling pathways exhibit antagonistic crosstalk with each other [35] , [36] . The ahg2-1 mutation enhances sensitivity to both phytohormones, a phenotype that has been rarely reported [22] . Our present study showed that this phenotype is caused by dysfunction of mitochondria, supporting the idea that mitochondria have roles in stress responses in plants [37] , [38] . In addition, given the ahg2-1 phenotype of abnormal crosstalk between ABA and SA, it is presumed that mitochondria are involved in the integration of various stress signals in plants. However, the linkage between plant hormonal responses and mitochondrial functions remains to be elucidated. The genetic resources of the AHG2–AGS1 system will be useful in addressing this missing link. PARN has been reported to be involved in vital biological functions through regulation of the poly(A) tract of cytoplasmic RNA in various organisms including plants [39] , [40] , [41] . As following this line, the recent report proposed that AHG2 negatively regulates post-transcriptional gene silencing in cytoplasm [33] . However, our present study surprisingly shows that PARN regulates the poly(A) status of mitochondrial mRNA in Arabidopsis . Plants have developed unique systems for the regulation of mitochondrial functions, and mitochondrial activity affects many aspects of fundamental physiological processes in plants, such as environmental stress responses and photosynthesis. Utilizing PARN as a regulator of mitochondrial mRNA stability represents another mechanism whereby plants control mitochondrial function. Plant material Arabidopsis thaliana (L.) Heynh. ecotypes Columbia (Col) and Landsberg erecta (L er ) were used in this work. Plants were grown on soil or on Murashige and Skoog (MS) plates containing 1 × MS salt mix, 2% sucrose, 2.5 mM MES (pH 5.8) and 0.8% agar. All sown seeds were first stratified at 4 °C for 4 days and then transferred to a growth chamber (22 °C with a 16-h light–8-h dark cycle), unless otherwise indicated. The AGS1 T-DNA insertion mutant line (SALK_083725) was obtained from TAIR [42] . Preparation of protoplasts and plasmid transfection were performed as described by Yoo et al . [43] Extraction and analysis of free SA was performed as described by Yasuda et al . [35] Ethyl methanesulfonate (EMS)-mutagenized M2 seeds were obtained as follows: ahg2-1 seeds were treated with 0.3% EMS for 16 h at room temperature (ca. 2000 seeds per parental group, using a total of eight parental groups), washed extensively with water, and sown on soil. M2 generation seeds were separately harvested and formed independent pools. For mapping the loci, the sup1 suppressor mutant was crossed with Ler wild type, and F2 progeny were obtained. Abscisic acid-hypersensitive individuals were selected on medium containing 0.2 μM ABA and grown on standard medium. In vitro polymerase assay Recombinant proteins were produced using the TNT SP6 high-yield wheat germ protein expression system (Promega KK, Tokyo, Japan) with halo-tag fused genes harboured by plasmid pFN19K, and then halo-tagged proteins were purified using the appropriate purification system (Promega) according to the manufacturer’s instructions. Template RNA was synthesized using pBluescript as described by Roberdatto et al . [19] Template RNA (0.4 μg) and recombinant proteins (~20 ng) were mixed and incubated in a buffer (HEPES (pH 7.2), 50 mM NaCl, 5 mM MgCl 2 , 1 mM DTT, 0.25 mM each ribonucleotide, total volume 10 μl) at 23 °C for 1 h. A portion (1 μl) of the reaction mixture was analysed using an Agilent Small RNA kit (Agilent Technologies, Tokyo, Japan) with an Agilent 2100 Bioanalyzer. cDNA synthesis and PAT assay Total RNA was isolated from plant materials using Sepasol reagent (Nacalai Tesque, Kyoto, Japan) and used for cDNA synthesis with a dT(15) + -T7 promoter sequence primer. PAT assays were performed using a cDNA mixture with the T7 primer and a gene-specific primer for the sequence near the 3′-end of mRNA ( Supplementary Table S3 ). As PAT assays using protoplast RNA gave higher background levels, it was difficult to estimate polyadenylated nad7 transcript levels via RT–qPCR. Therefore, PAT assay products were separated on agarose gels, and relative polyadenylated nad7 transcript levels were deduced from ethidium bromide fluorescence intensities using the signal intensity of a GFP-transfected protoplast sample as a control. The values were normalized to the endogenous ACT2 expression levels determined by RT–qPCR. The averages of the relative polyadenylated nad7 transcript levels with s.d.’s obtained from three independent transfection assays are presented. For each transfection, 2 × 10 5 cells were transfected with 100 μg of plasmid DNA. Total RNA was prepared from protoplasts 24 h after transfection and used for cDNA synthesis with a dT(15) + -T7 promoter sequence primer. The procedures for cRT–PCR were derived from Couttet et al . [44] ; gene-specific cRTR1 primers were used for cDNA synthesis after RNA circularization, and gene-specific cRTF and cRTR2 primers were used for PCR ( Supplementary Table S3 ). Microscopic observation Plant materials were stained with 100 nM of MitoTracker Red CMXRos (Life Technologies Corporation, Tokyo, Japan) for 15 min at room temperature and washed thrice with water (for roots) or WI buffer [43] (for protoplasts). Fluorescence was observed under a confocal microscope (FV1000-D; Olympus, Tokyo, Japan). Construction of transgenic plants For constructing transgenic plants, full genomic regions for AHG2 (Ch I NC_003070.9; 20,893,125–20,898,872 bp) and AGS1 (Ch II NC_003076.8; 7,644,456–7,650,515 bp) were obtained by PCR using gene-specific primers ( Supplementary Table S3 ). These genomic DNA segments included all exons and introns, and the upstream regions with part of the upstream gene. The nucleotide sequences of these clones were confirmed. The Venus GFP gene [45] was introduced into the Msc I site for AHG2 and into the Nde I site for AGS1 to generate fusion genes. The recombinant genes were introduced into pBI101 and used for generating transgenic Arabidopsis via Agrobacterium-mediated transformation [46] . To construct ΔN–AHG2 or ΔN–AGS1, the segment from 4–99 bp or 4–112 bp of the open reading frame was removed, respectively. For MtP–ΔN–AHG2 and MtP–ΔN–AGS1, the same regions were replaced with the segment from 4–321 bp of At5g14580 . Quantitative real-time PCR experiments Quantitative real-time PCR was performed on a LightCycler (Roche Diagnostics, Mannheim, Germany) in a total volume of 20 μl containing 10 μl SYBR Green Real-Time PCR Master Mix-Plus (Takara Bio Inc., Otsu, Japan), 8 pmol each primer and 1/40 of the cDNA mixture. The amplification program consisted of 40 cycles of 95 °C for 10 s and 60 °C for 1 min. The comparative C t method was used. For estimation of the relative amount of mt-DNA to nc-DNA, qPCR experiments for mitochondrial-encoded genes ( cox2 and nad4 ) and a nuclear-encoded gene ( AGS1 ) (primer sets: cox2F1–cox2R1, nad4F–nad4R and 17580F3–17580R1; Supplementary Table S3 ) were conducted using total DNA isolated from 2-week-old plants. For detection of polyadenylated nad7 transcripts, RT–qPCR was conducted using cDNA synthesized with dT(15) + -T7 promoter sequence primer as a template with two PCR primers (nad7pat and T7 primer, Supplementary Table S3 ). The relative polyadenylated transcript level was deduced with the comparative C t method using the expression of endogenous ACT2 as a control. For detection of mt-DNA or transcripts in purified mitochondria, total DNA or RNA was prepared from purified mitochondria. The volume or weight of mitochondria was estimated based on the total protein level quantified by the bicinchoninic acid method using the Pierce BCA Protein Assay Kit (Thermo Scientific, Rockford, Illinois, USA). cDNA was prepared from total mitochondrial RNA pretreated with ribonuclease-free DNase using random primers. Primers used for qPCR or qRT–PCR experiments are listed in Supplementary Table 3 . RNA gel blotting Total RNA was isolated from 3-week-old plants, separated on a 1.2% agarose gel, transferred to a nylon membrane and hybridized with DIG-labelled DNA probes. DNA labelling and detection were performed using a DIG High Prime DNA labelling and Detection Starter Kit II (Roche Diagnostics, Japan, Tokyo), following the manufacturer’s instructions. Purification of mitochondria and protein analysis Mitochondria were prepared from cultured plant cells obtained from callus induced from seedlings [34] . Cultured cells were disrupted in a blender in the presence of 0.3 M mannitol, 50 mM KH 2 PO 4 , 2 mM EGTA, 0.5% polyvinylpyrrolidone and 20 mM cysteine (pH 8.0) at 4 °C. After squeezing through nylon mesh (30 μm) the resultant homogenate was centrifuged at 2,000 g for 15 min at 4 °C, and the supernatant was centrifuged at 12,000 g for 15 min. The pellet was resuspended and used for purification of mitochondria using the Qproteome Mitochondria Isolation Kit (Qiagen KK, Tokyo, Japan). Mitochondrial proteins were solubilized with dodecylmaltoside (0.5 g per g of mitochondrial protein). BN–PAGE was performed using NativePAGE 4–16% gels (Life Technologies Japan, Ltd, Tokyo, Japan). For immunoblot analysis, proteins separated via SDS–PAGE or BN–PAGE were transferred to a PVDF membrane and exposed to primary antibodies against GFP (1:500 dilution), cox2 (1:1,000), CytC (1:1,000), cFBPase (1:5,000), nad9 (1:50,000), 51-kDa protein (1:1,000), SDH1 (1:1,000), αMPP (1:1,000), beta subunit (1:1,000) or Calnexin (1:5,000). Anti-GFP (No. 598) was purchased from MBL (Nagoya, Japan), and anti-cox2, -CytC and -cFBPase antisera were purchased from Agrisera (Viannas, Sweden). Anti-nad9 serum was a gift from Dr G. Bonnard (IBMP-CNS); anti-51-kDa protein, -SDH1, -αMPP and -beta subunit antisera were gifts from Dr K. Peters (Leibniz University, Hannover, Germany); anti-Calnexin was a gift from Dr F. Takaiwa (NIAS, Japan). How to cite this article: Hirayama T. et al . A poly(A)-specific ribonuclease directly regulates the poly(A) status of mitochondrial mRNA in Arabidopsis. Nat. Commun. 4:2247 doi: 10.1038/ncomms3247 (2013)